Attention gates visual coding in the human pulvinar The pulvinar nucleus of the thalamus is suspected to have an important role in visual attention, based on its widespread connectivity with the visual cortex and the fronto-parietal attention network. However, at present, there remain many hypotheses on the pulvinar's specific function, with sparse or conflicting evidence for each. Here we characterize how the human pulvinar encodes attended and ignored objects when they appear simultaneously and compete for attentional resources. Using multivoxel pattern analyses on data from two functional magnetic resonance imaging (fMRI) experiments, we show that attention gates both position and orientation information in the pulvinar: attended objects are encoded with high precision, while there is no measurable encoding of ignored objects. These data support a role of the pulvinar in distractor filtering—suppressing information from competing stimuli to isolate behaviourally relevant objects. The pulvinar nucleus of the thalamus is believed to have an important, integrative function in the mammalian brain, likely related to visual attention [1] , [2] . While pinpointing the pulvinar's specific role in vision has proven notoriously difficult, one line of evidence suggests the pulvinar may be important in isolating behaviourally relevant objects from surrounding distractors [3] , [4] , [5] , [6] , [7] . When Desimone et al . [5] deactivated the macaque pulvinar by muscimol injection, visual discrimination was impaired in the visual field contralateral to the injection site, but only when distractors were present; performance was unaffected in the absence of distractors. Recently [6] , a similar pattern was reported in human subjects with pulvinar lesions due to stroke: patients had compromised visual discrimination in the contralesional visual field, but only when salient distractors were present. These results point towards an involvement of the pulvinar in resolving competition between visual targets and distractors [8] , [9] . However, other studies based on lesions have failed to reinforce this notion. In a flanker interference task [10] and a global/local interference task [11] , subjects with pulvinar lesions showed no impairment in suppressing the distracting dimensions. These results reveal two missing pieces of the puzzle with regard to distractor filtering in the pulvinar. First, lesion studies still paint a mixed picture of whether intact pulvinar function is necessary for normal distractor suppression. This may be due partly to the wide variety of stimuli and tasks used across the studies. Second, and more importantly, the current evidence for the pulvinar's role in distractor suppression comes almost exclusively from monkey and human lesion studies. To establish a role of the human pulvinar in distractor suppression, it is critical to show that the pulvinar performs such a function in healthy humans. Here, we tested for distractor filtering in the human pulvinar by characterizing how the pulvinar encodes targets and distractors when they compete for attentional resources. We capitalize on a newly emerging understanding of the human pulvinar's organization [12] , [13] , [14] , [15] ; specifically, the presence of precise, lateralized spatial maps in both hemispheres. Using a multi-voxel pattern analysis, we measured the precision with which attended and ignored stimuli are coded in the pulvinar when both are present simultaneously within the same visual hemifield. Our results show that attention gates both spatial and featural information in the pulvinar: the positions and orientations of attended targets were coded with high precision in pulvinar responses, while there was no detectable encoding of distractor positions or orientations, even though the targets and distractors differed only in their behavioural relevance. These data support the hypothesis that the pulvinar is involved in filtering distracting visual information and highlighting behaviourally relevant targets. Attentional gating of spatial information in the pulvinar Subjects viewed four visual stimuli at a time; two were attended and two were ignored. The stimuli were Gabor patches in the four visual quadrants ( Fig. 1a ); in each 10-s stimulation block, they appeared at one of five possible eccentricities ranging from 8.4° to 9.6° ( Fig. 1b ). The top two Gabors were fixed to have the same eccentricity as each other, as were the bottom two, but the eccentricities for the upper and lower Gabors were random with respect to each other. On alternating runs, subjects attended to the Gabors in either the upper or the lower visual field ( Fig. 1c ), watching for slight contrast decrements that occurred an average of five times per block. Attention was manipulated between the upper and lower visual fields (rather than left versus right) so that an attended and an ignored stimulus were always present within the same visual field, and hence represented in the pulvinar in the same hemisphere. At the end of each block, the subject made a response indicating whether there were more contrast decrements on the left, right, or the same number on the left and right (3 AFC; sensitivity (d′) for the task was 1.59, indicating that the task was challenging but above threshold). The contrast decrements also occurred in the ignored stimuli, such that they were not just irrelevant but also distracting; subjects were motivated to ignore those stimuli as completely as possible. We tracked the eye positions of three of the five subjects during scanning ( Fig. 2 ). 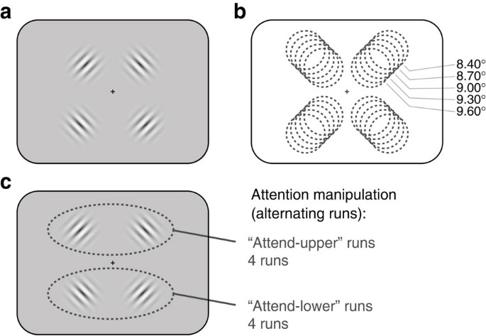Figure 1: Stimuli and experimental design. (a) The stimuli consisted of four Gabor patches in the four visual quadrants. (b) The Gabors appeared at five possible eccentricities, ranging from 8.40° to 9.60°. From trial to trial, the positions of the upper two Gabors varied independently of the positions of the lower Gabors. (c) In alternating runs, subjects were instructed to attend to the Gabors in either the upper visual field or the lower visual field, to detect slight contrast decrements in the stimuli. Figure 1: Stimuli and experimental design. ( a ) The stimuli consisted of four Gabor patches in the four visual quadrants. ( b ) The Gabors appeared at five possible eccentricities, ranging from 8.40° to 9.60°. From trial to trial, the positions of the upper two Gabors varied independently of the positions of the lower Gabors. ( c ) In alternating runs, subjects were instructed to attend to the Gabors in either the upper visual field or the lower visual field, to detect slight contrast decrements in the stimuli. 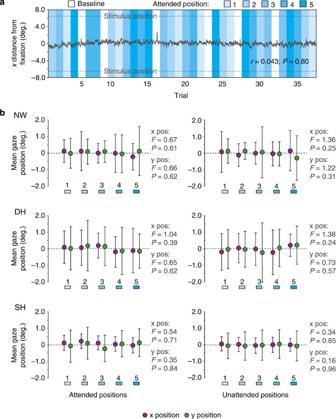Figure 2: Analysis of eye position data. (a) Example eye trace, showing the horizontal eye position across one run for subject DH. Shades of blue indicate the position of the attended stimuli on each trial. For this run, the correlation between mean horizontal eye position within each block and the stimulus eccentricity wasr=0.043 (P=0.80; based on 36 blocks per run; d.f.=34). The correlation between eye position and stimulus condition was not significant for any run, for either the attended or ignored stimuli. (b) Mean eye position is shown for each of the five attended positions and the five ignored positions separately for each subject. Error bars are the s.d. of the eye position measurements within each bin. We ran four one-way ANOVAs within each subject, testing for a systematic difference in horizontal or vertical eye position across the five stimulus locations for either the attended or ignored stimuli. None of these tests showed significant differences in eye position across the five stimulus locations (most significant was in subject DH for the ignored stimulus locations × horizontal eye position:F4,119995=1.38,P=0.24; allP-values reported reflect tests for a main effect of eye position across the five stimulus locations, with 120,000 total eye position measurements). These results rule out the influence of systematic eye movements on our results. Full size image Figure 2: Analysis of eye position data. ( a ) Example eye trace, showing the horizontal eye position across one run for subject DH. Shades of blue indicate the position of the attended stimuli on each trial. For this run, the correlation between mean horizontal eye position within each block and the stimulus eccentricity was r =0.043 ( P =0.80; based on 36 blocks per run; d.f.=34). The correlation between eye position and stimulus condition was not significant for any run, for either the attended or ignored stimuli. ( b ) Mean eye position is shown for each of the five attended positions and the five ignored positions separately for each subject. Error bars are the s.d. of the eye position measurements within each bin. We ran four one-way ANOVAs within each subject, testing for a systematic difference in horizontal or vertical eye position across the five stimulus locations for either the attended or ignored stimuli. None of these tests showed significant differences in eye position across the five stimulus locations (most significant was in subject DH for the ignored stimulus locations × horizontal eye position: F 4,119995 =1.38, P =0.24; all P -values reported reflect tests for a main effect of eye position across the five stimulus locations, with 120,000 total eye position measurements). These results rule out the influence of systematic eye movements on our results. Full size image Independently manipulating the positions of the upper and lower Gabors allowed us to separately measure position coding at the attended and ignored locations within the same functional run. We extracted patterns of blood oxygenation level-dependent (BOLD) responses corresponding to the attended and ignored stimuli from the same set of voxels by running two separate general linear models: one in which the five predictors were coded according to the positions of the attended stimuli, and one in which they were coded according to the positions of the ignored stimuli ( Fig. 3 ). In each general linear model (GLM), we separately contrasted the five predictors against the fixation baseline condition to obtain five maps of t -values. The result was a set of maps corresponding to the five attended positions and another set corresponding to the five ignored positions. Because the positions of the attended and ignored stimuli varied independently of each other, information about one of the dimensions was randomly distributed in the maps corresponding to the other dimension. Our subsequent pattern analysis tested for systematic variation in these activity maps as a function of stimulus position. 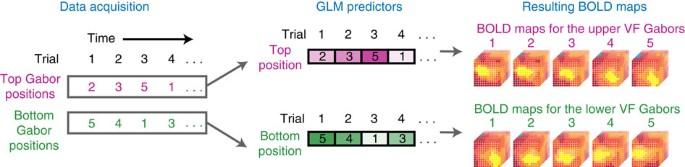Figure 3: Parallel analysis of the attended and ignored stimuli in the BOLD response. To separately isolate the patterns of activity corresponding to the attended stimuli and the ignored stimuli, we fit each functional run with two separate general linear models. One had predictors coded according to positions of the Gabors in the upper visual field (shown in purple), whereas the other had predictors coded according to positions of the Gabors in the lower visual field (shown in green). By separately contrasting each of the five stimulus positions against a fixation baseline in each GLM, we generated ten maps of BOLD response: five corresponding to positions of the stimuli in the upper visual field and five corresponding to the positions of the stimuli in the lower visual field. This approach allowed us to tease apart information about the attended and ignored stimulus positions within the same set of voxels by using two separate and independent encoding models, each of which explained a unique portion of the pattern of activity in the pulvinar ROI. Figure 3: Parallel analysis of the attended and ignored stimuli in the BOLD response. To separately isolate the patterns of activity corresponding to the attended stimuli and the ignored stimuli, we fit each functional run with two separate general linear models. One had predictors coded according to positions of the Gabors in the upper visual field (shown in purple), whereas the other had predictors coded according to positions of the Gabors in the lower visual field (shown in green). By separately contrasting each of the five stimulus positions against a fixation baseline in each GLM, we generated ten maps of BOLD response: five corresponding to positions of the stimuli in the upper visual field and five corresponding to the positions of the stimuli in the lower visual field. This approach allowed us to tease apart information about the attended and ignored stimulus positions within the same set of voxels by using two separate and independent encoding models, each of which explained a unique portion of the pattern of activity in the pulvinar ROI. Full size image We used a cross-correlation approach [16] , [17] , [18] , [19] , [20] to test for position selectivity in the BOLD response in the pulvinar. The analysis ( Fig. 4 ) tested whether stimuli presented closer together in space produced more similar patterns of activity. The centre (position 3) map was used as a baseline, and we compared the four other positions with it by cross-correlating the activity patterns ( Fig. 4a ). Cross-correlating all of the activity patterns for all stimulus positions against each other yielded similar results ( Supplementary Fig. S1 ), but using the central map as a baseline is more conservative because it avoids making assumptions about the linearity of the relationship between physical stimulus separation and correlation, as well as the independence of points in the plot ( Supplementary Methods ). In the plots in Fig. 4a , each point represents one voxel within the region of interest (ROI), its value from one BOLD map plotted on the x-axis ( t units), and its value from a second BOLD map plotted on the y-axis. The correlation across voxels between a given pair of BOLD maps served as a measure of their similarity within that ROI; we plotted the correlation between each pair as a function of the distance between the corresponding stimuli in visual space ( Fig. 4b ). A significant negative slope on this plot indicates precise discrimination of the stimulus positions—the multivariate pattern of response within the ROI in question changed systematically with changes in stimulus position. This analytical approach allowed us to separately measure the encoding of the attended and ignored stimuli within the pulvinar without making any assumption about the nature of the underlying topographic organization there. We performed this analysis in pulvinar ROIs defined based on the Talairach Atlas [21] , but fit to each subject's individual anatomy ( Fig. 4c ). 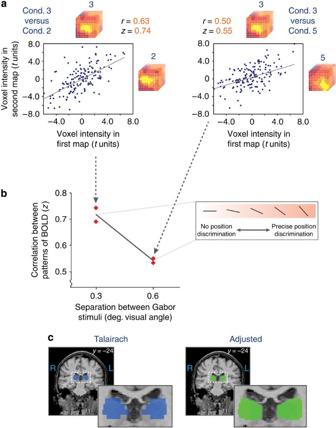Figure 4: Correlation-based analysis of position selectivity. (a) We computed the pairwise correlations between the patterns of activity produced by the five stimulus positions (the central condition versus each of the other conditions). Each point on the plot represents one voxel, its value from the first BOLD map plotted against its value from the second BOLD map. We then tested for a trend in the correlations indicating position selectivity by plotting them as a function of the visual distance between the corresponding stimuli (b). A negative trend in the plot of correlation values indicates that as the stimuli became more retinotopically distinct, they produced more distinct multivariate patterns of activity20. A steeper negative slope on the plot indicates more precise encoding of stimulus position. (c) To generate ROI for the pulvinar, we used the coordinates for the pulvinar drawn from the Talairach Atlas21(shown in blue), and made minor adjustments to match the ROIs to each subject's individual anatomy (an example of adjusted ROI is shown in green). Figure 4: Correlation-based analysis of position selectivity. ( a ) We computed the pairwise correlations between the patterns of activity produced by the five stimulus positions (the central condition versus each of the other conditions). Each point on the plot represents one voxel, its value from the first BOLD map plotted against its value from the second BOLD map. We then tested for a trend in the correlations indicating position selectivity by plotting them as a function of the visual distance between the corresponding stimuli ( b ). A negative trend in the plot of correlation values indicates that as the stimuli became more retinotopically distinct, they produced more distinct multivariate patterns of activity [20] . A steeper negative slope on the plot indicates more precise encoding of stimulus position. ( c ) To generate ROI for the pulvinar, we used the coordinates for the pulvinar drawn from the Talairach Atlas [21] (shown in blue), and made minor adjustments to match the ROIs to each subject's individual anatomy (an example of adjusted ROI is shown in green). 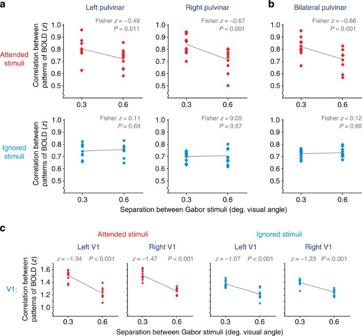Figure 5: Attention gates spatial encoding in the pulvinar. (a) Correlation-based analysis for left and right pulvinar, using the BOLD maps for the attended positions (red data) and the ignored positions (blue data). Each subject contributes four points to each plot—two independently computed correlations at each separation. Because multiple points were plotted for each subject, we fit the data with a regression model that included a random effect of subject22. Correlations are presented as Fisherz-scores for the sake of linear comparison. In both hemispheres, there was significant discrimination of the attended positions (Fisherz=−0.49,P=0.011 in left pulvinar;z=−0.67,P=0.001 in right pulvinar;n=20 for each test; non-parametric bootstrap test), but no discrimination of the ignored positions (z=0.11,P=0.69 in left pulvinar;z=0.05,P=0.57 in right pulvinar;n=20 for each test; non-parametric bootstrap test). (b) Position discrimination analysed in bilateral pulvinar ROIs. Discrimination of attended positions was significantly better than discrimination of ignored positions (P=0.01;n=20 points in each plot; bootstrap test for a difference in model fits between attended and ignored). (c) In primary visual cortex (V1), there was significant discrimination of both the attended and ignored stimulus positions, consistent with previous results20. Attentional modulation of position discrimination (zattended−zignored) was significantly greater in the pulvinar than in V1 (P=0.04;n=20 points in each plot; bootstrap test for a greater attended–ignored difference in the pulvinar versus V1). Full size image Figure 5a shows position discrimination for attended objects (red data) and ignored objects (blue data) in the pulvinar. Data from the five subjects are plotted together and fit with a regression model that included a random effect of subject [22] . Both the left and right pulvinar showed significant coding of the attended stimulus positions, as indicated by significant negative slopes in the regression fits (Fisher z =−0.49, P =0.011 in left pulvinar and z =−0.67, P =0.001 in right pulvinar; n =20 for each test; P -values were assessed using a non-parametric bootstrap test described in the Methods). All subjects showed the same trend individually. However, there was no detectable encoding of ignored objects ( z =0.11 in left pulvinar and z =0.05 in right pulvinar, both P >0.5; n =20 for each test; non-parametric bootstrap test). Figure 5b shows the same analysis performed in bilateral pulvinar ROIs; discrimination of attended positions was significantly better than discrimination of ignored positions ( P =0.01; n =20 points in each plot; bootstrap test for a difference in model fits between attended and ignored). It is important to note that the data in the attended and ignored plots came from the same functional runs, analysed within the same set of voxels, with the same stimuli present; no difference in signal-to-noise ratio, retinotopically specific adaptation, or other aspects of signal quality could explain the difference in coding precision we found for attended and ignored objects in the pulvinar ( Supplementary Methods ). These data demonstrate an essentially absolute gating of spatial information in the pulvinar by attention: only attended positions are encoded in the multi-voxel pattern of activity within the pulvinar. Figure 5: Attention gates spatial encoding in the pulvinar. ( a ) Correlation-based analysis for left and right pulvinar, using the BOLD maps for the attended positions (red data) and the ignored positions (blue data). Each subject contributes four points to each plot—two independently computed correlations at each separation. Because multiple points were plotted for each subject, we fit the data with a regression model that included a random effect of subject [22] . Correlations are presented as Fisher z -scores for the sake of linear comparison. In both hemispheres, there was significant discrimination of the attended positions (Fisher z =−0.49, P =0.011 in left pulvinar; z =−0.67, P =0.001 in right pulvinar; n =20 for each test; non-parametric bootstrap test), but no discrimination of the ignored positions ( z =0.11, P =0.69 in left pulvinar; z =0.05, P =0.57 in right pulvinar; n =20 for each test; non-parametric bootstrap test). ( b ) Position discrimination analysed in bilateral pulvinar ROIs. Discrimination of attended positions was significantly better than discrimination of ignored positions ( P =0.01; n =20 points in each plot; bootstrap test for a difference in model fits between attended and ignored). ( c ) In primary visual cortex (V1), there was significant discrimination of both the attended and ignored stimulus positions, consistent with previous results [20] . Attentional modulation of position discrimination ( z attended − z ignored ) was significantly greater in the pulvinar than in V1 ( P =0.04; n =20 points in each plot; bootstrap test for a greater attended–ignored difference in the pulvinar versus V1). Full size image If the attentional gating of spatial information we observed in the pulvinar is related to filtering out distractors, we would expect measurable encoding of the ignored stimulus positions at earlier stages of visual processing, including in the input signals to the pulvinar. We repeated the same analysis in seven independently localized visual areas: V1, V2, V3, V3a, VP, V4v and MT+. Figure 5c shows position discrimination plots, constructed in the same way as those shown for the pulvinar, for V1: V1 exhibited precise coding of both the attended and the ignored stimuli (attended: left- z =1.34, right- z =1.46; ignored: left- z =1.07, right- z =1.23; all P <0.001; n =20 for each test; non-parametric bootstrap test). In contrast to the pulvinar, each of the seven comparison visual areas showed significant discrimination of the ignored stimulus positions (non-parametric bootstrap test with n =20 for each test; all P <0.02; significant with FDR control for multiple comparisons [23] with q =0.05). Only the pulvinar displayed a complete gating of the ignored object positions, and attentional modulation of position coding was significantly stronger in the pulvinar than in the visual cortex ( P =0.008; n =20 points in each plot; bootstrap test for a greater attended–ignored difference in the pulvinar versus visual cortex). Of particular note is the significant encoding of ignored positions in MT+, which is thought to have a high density of driving input to the pulvinar [24] . Attentional gating of orientation information in the pulvinar We sought to test whether attention gates types of stimulus information besides position coding in the pulvinar. We also sought to verify that attentional gating in the pulvinar happens for task-relevant stimulus features (in experiment 1, subjects attended at the locations of the cued stimuli, but were not required to make a position-related judgment). Three subjects participated in this second experiment. The experimental design was similar to the first experiment, but now subjects were required to detect orientation changes in the cued Gabors. Each Gabor was oriented at either −45° or +45° relative to vertical, and the orientations in the upper and lower visual fields varied independently of each other from block to block ( Fig. 6a ). The left and right Gabors within the upper or lower visual field always had opposite orientations. An average of eight times per block, one of the four Gabors changed in orientation by 8°., for 200 ms. At the beginning of each run, subjects were instructed to attend to the orientations of either the upper two or lower two Gabors, and respond any time they detected an orientation change in one of the cued Gabors but to ignore orientation changes in the other two. Sensitivity (d′) for the orientation change detection task was 1.15; the task was challenging but above threshold. 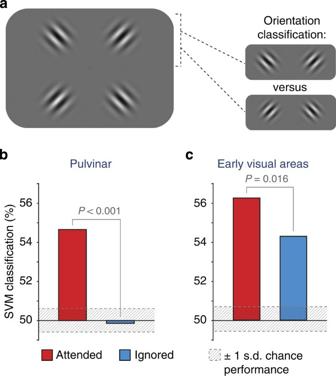Figure 6: Attention gates orientation encoding in the pulvinar. (a) Stimuli for the orientation decoding experiment. Gabor patches were presented in the four visual quadrants; the Gabors could be oriented at −45° or +45° with respect to vertical, and the orientations in the upper and lower visual fields varied independently (left and right Gabors within the upper or lower visual field were always oriented orthogonally). Subjects attended for brief orientation changes in the cued Gabors, ignoring the others. (b) Classification of attended and ignored orientations within the pulvinar. ±1 s.d. of chance classification, estimated by classifying with shuffled labels, is shown by the shaded region (Supplementary Methods). There was reliable classification of attended orientations (red bar; 54.7% correct; 7.8 s.d. above the mean of the bootstrapped chance distribution;P<0.001), but chance classification of ignored orientations (blue bar; 49.9% correct; 0.34 standard deviations below bootstrapped chance;P=0.62) in the pulvinar (n=192 training blocks and 48 test blocks per subject for both tests; data shown are collapsed across three subjects). Classification of attended orientations was significantly better than classification of ignored orientations (P<0.001; non-parametric bootstrap test for whether the attended-chance difference was larger than the ignored-chance difference;n=192 training blocks and 48 test blocks per subject in each condition). (c) In early visual areas (V1 through MT+), orientation classification was significantly above chance for both attended and ignored Gabors (56.3% correct for attended and 54.3% correct for ignored, 10.1 and 6.8 s.d. above bootstrapped chance, respectively; bothP<0.001;n=192 training blocks and 48 test blocks per subject for both tests). Attended orientations were classified significantly better than ignored orientations in early visual areas (P=0.016; bootstrap test for (attended-chance) > (ignored-chance)), but the modulation of orientation coding by attention was significantly stronger in the pulvinar than in early visual areas (P=0.012; bootstrap test for (pulvinarattended−pulvinarignored) > (early visattended−early visignored);n=192 training blocks and 48 test blocks per subject per condition for both tests). Figure 6: Attention gates orientation encoding in the pulvinar. ( a ) Stimuli for the orientation decoding experiment. Gabor patches were presented in the four visual quadrants; the Gabors could be oriented at −45° or +45° with respect to vertical, and the orientations in the upper and lower visual fields varied independently (left and right Gabors within the upper or lower visual field were always oriented orthogonally). Subjects attended for brief orientation changes in the cued Gabors, ignoring the others. ( b ) Classification of attended and ignored orientations within the pulvinar. ±1 s.d. of chance classification, estimated by classifying with shuffled labels, is shown by the shaded region ( Supplementary Methods ). There was reliable classification of attended orientations (red bar; 54.7% correct; 7.8 s.d. above the mean of the bootstrapped chance distribution; P <0.001), but chance classification of ignored orientations (blue bar; 49.9% correct; 0.34 standard deviations below bootstrapped chance; P =0.62) in the pulvinar ( n =192 training blocks and 48 test blocks per subject for both tests; data shown are collapsed across three subjects). Classification of attended orientations was significantly better than classification of ignored orientations ( P <0.001; non-parametric bootstrap test for whether the attended-chance difference was larger than the ignored-chance difference; n =192 training blocks and 48 test blocks per subject in each condition). ( c ) In early visual areas (V1 through MT+), orientation classification was significantly above chance for both attended and ignored Gabors (56.3% correct for attended and 54.3% correct for ignored, 10.1 and 6.8 s.d. above bootstrapped chance, respectively; both P <0.001; n =192 training blocks and 48 test blocks per subject for both tests). Attended orientations were classified significantly better than ignored orientations in early visual areas ( P =0.016; bootstrap test for (attended-chance) > (ignored-chance)), but the modulation of orientation coding by attention was significantly stronger in the pulvinar than in early visual areas ( P =0.012; bootstrap test for (pulvinar attended −pulvinar ignored ) > (early vis attended −early vis ignored ); n =192 training blocks and 48 test blocks per subject per condition for both tests). Full size image We measured orientation coding within the pulvinar and visual cortex separately for the attended and ignored stimuli, which were simultaneously present at all times. To measure orientation coding, we used a support vector machine (SVM) pattern classifier to predict which orientation had been presented on each block. We used SVM in the second experiment rather than the correlation analysis because the power of the latter is diminished when discriminating between just two stimulus categories rather than a multi-level parametric stimulus manipulation (in the analysis of the first experiment, though we paired stimuli according to two possible separations, we utilized all five stimulus conditions); SVM, however, is well suited to this case of binary classification [25] . Classification results are shown for the pulvinar and early visual cortex in panels b and c of Fig. 6 , respectively (data are collapsed across the three subjects). In the pulvinar, we found robust encoding of the attended stimulus orientations (54.7% correct; P <0.001; 7.8 s.d. above the mean of the bootstrapped chance distribution; n =192 training blocks and 48 test blocks per classification iteration per subject; reported performance is an average across 1,000 classification iterations) but no evidence of encoding of ignored orientations (49.9% correct; P =0.62; 0.34 s.d. below bootstrapped chance; n =192 training blocks and 48 test blocks per subject). Classification of the attended orientations was significantly better than classification of ignored orientations ( P <0.001; non-parametric bootstrap test for whether the attended-chance difference was larger than the ignored-chance difference; n =192 training blocks and 48 test blocks per subject in the classification of both the attended and ignored stimulus orientations). In the visual cortex, in contrast to the pulvinar, we found significant classification of both attended and ignored stimulus orientations (56.3% correct for attended and 54.3% correct for ignored, 10.1 and 6.8 s.d. above bootstrapped chance, respectively; both P <0.001; n =192 training blocks and 48 test blocks per subject). Consistent with previous findings [26] , [27] , [28] , attended orientations were classified significantly better than ignored orientations in early visual areas ( P =0.016; bootstrap test for (attended-chance) > (ignored-chance); n =192 training blocks and 48 test blocks per subject per condition). Importantly, the modulation of orientation coding by attention was significantly stronger in the pulvinar than in early visual areas ( P =0.012; bootstrap test for (pulvinar attended −pulvinar ignored ) > (early vis attended −early vis ignored ); n =192 training blocks and 48 test blocks per subject per condition). These results demonstrate that attention gates not only spatial representations but also orientation information within the pulvinar. They also demonstrate attentional gating of a task-relevant feature within the pulvinar. Collectively, our results show a gating of ignored information within the pulvinar that generalizes across at least two stimulus features (position and orientation) and is distinct from the pattern of attentional modulation we observed in the visual cortex. Our results show that stimulus encoding in the human pulvinar is gated by attention: when behaviourally relevant visual stimuli compete with distractors for attentional resources within the same visual field, the pulvinar precisely represents attended but not ignored objects. Thus, activity in the pulvinar reflects an isolated representation of attended targets, which can serve to selectively confer further processing benefits on important stimuli. Previous studies [12] , [14] , [29] have reported significant functional magnetic resonance imaging (fMRI) responses in the pulvinar to unattended stimuli. For example, when Smith et al . [29] presented subjects with optic flow stimuli and examined the BOLD response in the pulvinar when attention was directed either towards or away from the stimuli, they found significant pulvinar activation in both the attended and unattended cases, with an ∼ 20% amplitude modulation with attention. How do our present results square with these previous findings? First, it is important to distinguish between the amplitude of the raw BOLD response and information content in fMRI patterns of activity, which can be dissociated [26] , [30] , [31] ; our study takes the important step of decoding position and orientation information within the multivariate pattern of activity in the pulvinar, providing converging evidence for attentional gating from two information-based MVPA approaches. Equally important, though, is a key difference in experimental design between the above-mentioned studies and our study. The spatial attention manipulations in both Smith et al . [29] and Schneider [12] had attended and ignored stimuli on opposite sides of the horizontal meridian, and thus in different hemispheres in the pulvinar. Given the evidence for at least partially independent attentional resources in the left and right hemispheres [32] , [33] , one possibility is that a left/right attentional manipulation induces less competition between attended and unattended stimuli than if both stimuli fell in the same visual field. Thus, a key aspect of our design is the upper/lower manipulation of attention, forcing targets and distractors to compete for attentional resources within the same visual field and same hemisphere. Previously [13] , we reported position sensitivity in the pulvinar under passive viewing conditions (attention was engaged at the fixation point by a task unrelated to the stimuli). Critically, the stimuli used to measure spatial discrimination were neither targets nor distractors—they were irrelevant to the fixation task that subjects performed. Other studies of retinotopy in the healthy human pulvinar have used undivided attention [14] , [15] or featural attention [12] , but our study is the first to test how the healthy human pulvinar responds to competing stimuli in the same visual field. We introduced competition between simultaneously presented stimuli, which resulted in the ignored objects being gated out from encoding in the pulvinar. Unlike putative attentional source regions such as the IPS areas [34] , which show only weak responses to passive visual stimulation, the pulvinar precisely encodes passively viewed stimuli [13] but not distracting ones. We intentionally analysed ROIs that encompassed the entire pulvinar. Although the primate pulvinar has been classically divided into several subnuclei based on cytoarchitecture [35] , no structural or functional homology between the monkey and human pulvinars has been firmly established [6] . Further, interactions between attentional signals and visual maps in the pulvinar likely involve more than a single subregion. While the lateral and inferior portions of the monkey pulvinar are the most visually responsive [1] , [36] , the pulvinar's connections with areas in the fronto-parietal attention network project from the medial portion [37] . We therefore considered the multivariate pattern of activity within the pulvinar as a whole. Our results dovetail with recent reports that visual awareness is correlated with variability in the strength of responses in the pulvinar [38] , [39] . For example, Padmala et al . [38] used affective conditioning to increase the salience of otherwise neutral stimuli. Then, presenting conditioned and non-conditioned stimuli in a rapid serial visual presentation task during scanning, they found that stimulus detection was correlated with larger responses in the pulvinar; this effect was much larger for affectively conditioned stimuli. Our present results are complementary and demonstrate the flip side of the coin: we show that distracting stimuli are gated out from encoding in the pulvinar, while Padmala et al . demonstrated that the more salient an attended target is, the more robust a response it produces in the pulvinar, particularly if it has conditioned affective significance. In future work, it will be important to study whether and how affective significance interacts with the attentional gating effect we report here. Our orientation classification results complement and extend previous work on decoding orientation information from the human visual cortex [26] , [27] , [28] . Earlier work has shown that attending to an orientation biases signals in the visual cortex to preferentially represent that orientation, yielding a boost in classification accuracy [27] , [28] . This attention-related enhancement can occur selectively for task-relevant features [26] , and is carried at least in part by a boosted response within the subpopulation of voxels that is tuned to the attended orientation [27] . In experiment 2, we similarly found that attention significantly improved the precision of orientation coding in early visual cortex ( Fig. 6c ). We extended the classification framework to measure orientation-selective responses in the human pulvinar for the first time, and found a significantly larger attentional modulation of orientation information in the pulvinar than in the visual cortex ( Fig. 6b ), such that there was no measurable information about the ignored orientations, even though the ignored and attended stimuli differed only in their task relevance. The gating of orientation information in the pulvinar by attention sets the pulvinar apart from the pattern of results found in the visual cortex, and lends support to the hypothesis that the pulvinar has an important role in distractor filtering. Selective attention reduces the deleterious influences of distracting information on perception and behaviour, [9] , [40] , [41] , [42] and is therefore a critical mechanism for many visuomotor and cognitive functions. The pulvinar has long been suspected to be a neural interface where attention signals can gate out distractors, but this filtering function has never been observed in action in the pulvinar. Our results show that in the healthy human pulvinar, visual distractors are gated out from spatial coding, leaving a map that can serve to isolate behaviourally relevant objects and their features from among competing information. Subjects Seven healthy subjects, ranging in age from 22 to 31 years, participated in the study. All subjects provided written consent before participation, and all experimental procedures were approved by the UC Davis and UC Berkeley institutional review boards. Experimental design Before each scanning run, subjects were cued to attend to the Gabors in either the upper or lower visual field, and the subject attended at that location for the duration of the entire run. Attend-upper and attend-lower runs were interleaved so that no trends across the scanning session could differentially affect the two conditions. Within a run, the Gabor positions in the upper and lower visual fields were random with respect to each other, and the ordering of the conditions within the upper and lower visual fields was pseudo-randomized by shuffling within a group of the five position conditions plus a baseline condition, and then presenting six such shuffled groups in sequence. The Gabors (0.4 cycles per degree, peak contrast 87% (Michelson), 1.66°. s.d. envelope, 8 Hz counterphase flicker) appeared at five possible eccentricities, ranging from 8.40° to 9.60° in increments of 0.3°. Attend-upper and attend-lower runs were constructed in a completely identical fashion; the only difference between the two run types was the attended location. This upper/lower attention manipulation allowed the positions of the attended and ignored Gabors to vary independently of each other, and for both attended and ignored stimuli to be represented in each hemisphere. Stimuli were presented in 10-s blocks. We used a blocked design, rather than a rapid event-related design, to maximize the power in the position discrimination analysis ( Supplementary Methods ). In experiment 2, we measured orientation discrimination rather than position discrimination. Subjects viewed four Gabors (0.4 cycles per degree, 87% peak Michelson contrast, 1.66°. s.d. envelope, 8 Hz counterphase flicker), one in each visual quadrant ( Fig. 6a ). The orientations of the Gabors in the upper and lower visual fields varied independently ( Fig. 6a ), and the positions of the Gabors were randomly jittered from block to block with a s.d. of 0.47° (mean 9.0° eccentricity), independently in the upper and lower visual fields and independently of the orientations, to ensure that orientation decoding generalized across changes in position and was not simply capitalizing on localized luminance differences between orientations. Successful performance on the orientation change detection task required attending to both Gabors in the cued location (upper or lower visual field), while ignoring the Gabors in the non-cued field as completely as possible. As in experiment 1, the stimuli in attend-upper and attend-lower runs were constructed in a completely identical fashion; the only difference was the verbal instruction at the beginning of the run. fMRI acquisition Scanning was conducted on a Siemens Trio 3T system at the UC Davis Imaging Research Center. Functional images were collected with a gradient-recalled echo EPI sequence using an eight-channel phased-array head coil. Whole-brain anatomical images were acquired with a high-resolution (1 mm 3 ) Turbo Spin Echo scan. The acquisition parameters were: TR=2,000 ms, TE=26 ms, FA=90°, FOV=22×22 cm 2 , voxel size=1.528×1.528×2.5 mm 3 . The 24-slice imaging volume was centred on the thalamus and ran through the occipital pole. Runs were 360 s long (180 volumes). Using a Digital Projection Mercury 5000HD projector, stimuli were back-projected at 75 Hz onto a semi-transparent screen from outside the bore. Subjects were able to see the screen and stimuli via a mirror angled at 45°, located 9.5 cm directly above their eyes. Each subject participated in eight main experimental runs and one additional retinotopic localizer run. Data analysis fMRI data preprocessing, ROI definition and general linear models were performed in BrainVoyager QX v. 2.0; all other analysis was performed in Matlab R2008a. Data preprocessing consisted of slice scan time correction with cubic spline interpolation, 3D motion correction with trilinear interpolation and high-pass filtering with a cutoff of two cycles per run. The data were not otherwise spatially smoothed. The data were normalized to Talairach space to allow for atlas-assisted definition of the pulvinar ROIs ( Fig. 4c ). Position discrimination For each functional run, we constructed two general linear models, one with the five attended stimulus positions as five predictors, and the other with the five ignored stimulus positions as predictors. In addition, there was a sixth predictor for the baseline (fixation only) blocks. Figure 3 depicts the GLM recoding procedure. For each GLM, we separately contrasted each of the five stimulus position predictors against the fixation baseline to generate five maps of BOLD response ( t values) for use in the correlation analysis ( Fig. 4 ). In the group analysis of position discrimination, we used a random effects model to account for between-subject variability [22] . The regression model took the form z ijk = β 0 + βx jk + U i + ɛ ijk , where i indexed the subjects, the pair ( j , k ) indexed the stimulus pairings, and U i accounted for intercept differences between subjects. This approach is comparable to a paired t -test and yields identical P -values; we express the model in the general regression framework to make clear how the random effect of subject is incorporated into the model, and to visualize the slope of the data across stimulus separations. For significance testing, we generated bootstrapped confidence intervals for the group regression by sampling with replacement within each subject on 2,000 iterations ( Supplementary Methods ). Orientation discrimination To measure the encoding of orientation information in the pulvinar and visual cortex, we used a SVM classification analysis implemented in Matlab using the LIBSVM library [43] . Classification was run on block-by-block beta weights, rather than the raw BOLD timecourse, to improve SNR in the classification and account for hemodynamic lag. Within each subject and each ROI, we concatenated the blockwise beta maps from all runs, and ran 1,000 iterations of SVM classification with a linear kernel, each time training on a randomly selected 80% of blocks and testing on the remaining 20%. Overall classification accuracy was taken as the average classifier performance across the 1,000 classification iterations. A label-shuffling procedure confirmed that the training process did not 'peek' at the test data ( Supplementary Methods ). ROI definition No functional localizer exists for the pulvinar, and portions of the pulvinar can be difficult or impossible to delineate based on anatomical scans alone. Because of this, we based our pulvinar ROI definitions on standardized coordinates drawn from the Talairach Atlas [21] . To define individual pulvinar ROI for each subject, we began with standard pulvinar ROI drawn from the Talairach atlas (shown in blue in Fig. 4c ), and made minor manual corrections based on each subject's anatomy. Corrections were only made where the atlas-based ROIs encroached on ventricle space or clearly disobeyed grey/white matter boundaries. We used the coronal plane running through the posterior commissure as a conservative anterior boundary to ensure that no grey matter outside the pulvinar was included the ROIs. The result was a left- and right-pulvinar ROI for each subject that fit the individual anatomy while staying close to the atlas coordinates (example ROIs shown in green in Fig. 4c ). To localize the early retinotopic visual areas in each subject, subjects participated in a separate scanning run consisting of standard localizer stimuli including flickering checkerboard wedge and drifting stimuli presented along the horizontal and vertical meridians [44] . A map that contrasted the horizontal and vertical meridians was overlaid on an inflated surface map for each subject, and the meridians were used to delineate the early retinotopic areas. How to cite this article: Fischer, J. & Whitney, D. Attention gates visual coding in the human pulvinar. Nat. Commun. 3:1051 doi: 10.1038/ncomms2054 (2012).